Regulation of the DNA damage response on male meiotic sex chromosomes During meiotic prophase in males, the sex chromosomes partially synapse to form the XY body, a unique structure that recruits proteins involved in the DNA damage response, which is believed to be important for silencing of the sex chromosomes. It remains elusive how the DNA damage response in the XY body is regulated. Here we show that H2AX-MDC1-RNF8 signaling, which is well characterized in somatic cells, is dispensable for the recruitment of proteins to the unsynapsed axes in the XY body. On the other hand, the DNA damage response that spreads over the sex chromosomes is largely similar to that in somatic cells. This analysis shows that there are important differences between the regulation of the DNA damage response at the XY body and at DNA damage sites in somatic cells. Meiotic prophase is one of the most important stages before meiotic divisions in both male and female reproductive germ cells. During this period, homologous chromosomes synapse and undergo meiotic recombination. The exchange of genetic material between homologous chromosomes is critical for generating genetic diversity in the offspring. Meiotic recombination starts with global SPO11-dependent DNA breaks throughout the chromosomes, which trigger the DNA damage response (DDR) [1] . Meiotic recombination occurs during chromosome synapsis, when DNA repair takes place through homologous recombination. One unique challenge during male meiosis is that male spermatocytes possess X and Y sex chromosomes, which are largely heterologous and only partially synapse through their pseudo autosomal regions. When autosomes are fully synapsed and meiotic recombination is finished at pachynema of meiotic prophase, DDR proteins are lost from the autosomes and autosomes become transcriptionally active. However, the partially synapsed sex chromosomes at pachynema locate to a region close to the edge of the nucleus known as the XY body, and remain transcriptionally silenced. This phenomenon is known as meiotic sex chromosome inactivation (MSCI) (ref. 2 ). It is known that the XY body retains a lot of DDR proteins, which are believed to be important for the initiation of MSCI. Consistent with this idea, spermatocytes deficient for H2AX or MDC1, two proteins that act early in the DDR pathway in somatic cells, abolished MSCI (refs 3 , 4 ). Although many DDR proteins accumulate in the XY body, their localizations are different [4] . Some proteins, such as H2AX and MDC1, spread over the sex chromosomes. Some proteins, like ATR and TopBP1, are more concentrated at the unsynapsed axes, and are weakly stained on the sex chromosomes. Some proteins, including BRCA1, are exclusively located at the unsynapsed axes. In addition, single-stranded DNA-binding protein RPA and DNA repair protein RAD51 form foci specifically at the unsynapsed axes. This suggests that the unsynapsed axes are different from other chromosomal regions of the XY body, and that the regulation of DDR in spermatocytes could be distinct from that in somatic cells. Recent studies have suggested that the DDR begins by recruiting some proteins to the unsynapsed axes in a MDC1-independent manner. This is then followed by MDC1-dependent amplification of the DDR to other regions of the sex chromosomes [4] . RNF8 is a protein immediately downstream of MDC1 in the DDR in somatic cells [5] , [6] . Different from Mdc1 knockout spermatocytes that arrest at mid-pachynema without proper formation of the XY body, meiosis in Rnf8 knockout mice progresses normally and the XY body forms readily in spermatocytes at pachynema [7] . Therefore, Rnf8 knockout mice are better tools for examining the DDR signalling at the meiotic sex chromosomes in the XY body. In this study, we analyse the DDR signalling of the XY body in Rnf8 knockout spermatocytes and explore potential mechanisms that recruit the DDR proteins to the unsynapsed axes. We find that there are important differences between the regulation of the DDR at the XY body and at DNA damage sites in somatic cells. RNF8 controls DDR protein localization on sex chromosomes Consistent with our prior observations, RNF8 deficiency has no obvious impact on meiotic prophase, and spermatocytes still progress through pachynema with normal XY body formation. RNF8 is known to be essential for protein ubiquitination in the XY body ( Fig. 1a ; ref. 7 ). To distinguish which ubiquitin species is enriched in the XY body, we tested antibodies that specifically recognize K48 or K63-linked ubiquitin chains [8] . In agreement with the well-characterized observation that RNF8 promotes the synthesis of K63-linked ubiquitin chains at DNA damage sites in somatic cells [9] , K63-linked ubiquitination was enriched in the XY body and was absent in Rnf8 knockout spermatocytes ( Fig. 1b ). Recent studies have shown that RNF8 also facilitates the transient assembly of K48-linked ubiquitin chains at DNA damage sites in somatic cells [10] , [11] . Interestingly, K48-linked ubiquitination was also enriched in the XY body of wild-type, but not Rnf8 knockout spermatocytes ( Fig. 1c ). These results suggest that RNF8 regulates both K48 and K63-linked ubiquitination in the XY body. Besides ubiquitination, sumoylation is another ubiquitination-like protein modification at DNA damage sites [12] , [13] . It has been shown that RNF8 is important for protein modification by SUMO1 or SUMO2/3 at DNA damage sites [13] , and both of them have been shown to enrich in the XY body and spread over the sex chromosome [14] . Interestingly, we found that both SUMO1 and SUMO2/3 still localized to the XY body in Rnf8 knockout spermatocytes ( Fig. 1d ). Therefore, RNF8 is dispensable for protein sumoylation in the XY body, which is different from the DDR in somatic cells. 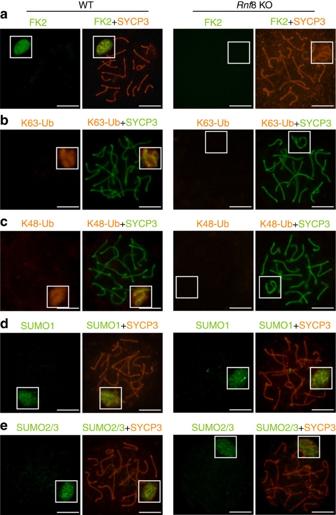Figure 1: RNF8 controls protein ubiquitination but not sumoylation in the XY body. Spermatocytes at pachynema from WT andRnf8knockout mice were stained using antibodies against ubiquitin-FK2 (a), K63-linked ubiquitin chains (b), K48-linked ubiquitin chains (c), SUMO1 (d) and SUMO2/3 (e). SYCP3 was used to visualize the chromosome synapsis and to differentiate spermatocytes at various stages of meiotic prophase. Scale bar, 10 μm. Figure 1: RNF8 controls protein ubiquitination but not sumoylation in the XY body. Spermatocytes at pachynema from WT and Rnf8 knockout mice were stained using antibodies against ubiquitin-FK2 ( a ), K63-linked ubiquitin chains ( b ), K48-linked ubiquitin chains ( c ), SUMO1 ( d ) and SUMO2/3 ( e ). SYCP3 was used to visualize the chromosome synapsis and to differentiate spermatocytes at various stages of meiotic prophase. Scale bar, 10 μm. Full size image As RNF8 is important for propagating DNA damage signals and controls the localization of a number of proteins at DNA damage sites in somatic cells, we examined if RNF8 deficiency has any impact on the localization of a number of DDR proteins in spermatocytes. Proteins in somatic DDR pathways upstream of RNF8 (H2AX and MDC1) were still enriched in the XY body and spread over the sex chromosomes in Rnf8 knockout spermatocytes ( Fig. 2a ). It is well characterized that 53BP1 is downstream of RNF8 in the DDR of somatic cells [5] , [6] . 53BP1 was localized at the XY body and spread over the sex chromosomes in wild-type spermatocytes, but was absent in Rnf8 knockout spermatocytes ( Fig. 2c ). Although how RNF8 regulates 53BP1 in somatic DDR is not clear, it seems that it regulates 53BP1 using the same mechanism in spermatocytes. It is also known that the RNF8-dependent ubiquitin chains directly recruit RAD18 to DNA damage sites in somatic cells [15] , and RAD18 spreads over the sex chromosomes [16] . Interestingly, the localization of RAD18 to the XY body was completely abolished in Rnf8 knockout spermatocytes, which is consistent with the absence of ubiquitin chains ( Fig. 2d ). As the absence of both 53BP1 and RAD18 in the XY body does not affect the meiosis of Rnf8 knockout spermatocytes, these two proteins are likely dispensable for meiosis, which is consistent with previous studies of mice lacking either of them [17] , [18] , [19] . Besides proteins that spread over the sex chromosomes, some proteins in the XY body, like ATR and TopBP1, spread over the sex chromosomes with enrichment in the unsynapsed axes [20] . In agreement with the observation that RNF8 deficiency does not affect ATR or TopBP1 foci in somatic cells [21] , there was little difference in the localizations of ATR or TopBP1 between wild-type and Rnf8 knockout spermatocytes ( Fig. 2e ). Although it has been suggested that MDC1 is required for the spread of ATR and TopBP1 over the sex chromosomes [4] , RNF8 seems to be dispensable for this process. 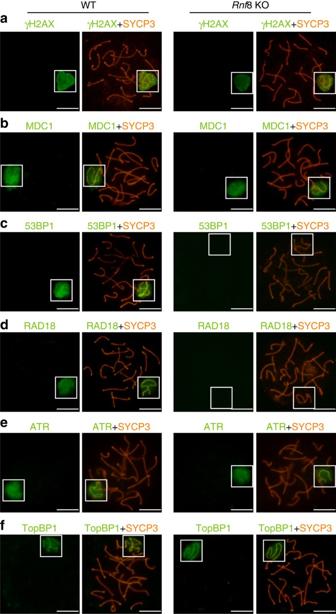Figure 2: RNF8 controls the localization of DDR proteins over the sex chromosomes. Spermatocytes at pachynema from WT andRnf8knockout mice were stained using the antibodies antibodies against γH2AX (a), MDC1 (b), 53BP1 (c), RAD18 (d), ATR (e) and TopBP1 (f). SYCP3 was used to visualize the chromosome synapsis and to differentiate spermatocytes at various stages of meiotic prophase. Scale bar, 10 μm. Figure 2: RNF8 controls the localization of DDR proteins over the sex chromosomes. Spermatocytes at pachynema from WT and Rnf8 knockout mice were stained using the antibodies antibodies against γH2AX ( a ), MDC1 ( b ), 53BP1 ( c ), RAD18 ( d ), ATR ( e ) and TopBP1 ( f ). SYCP3 was used to visualize the chromosome synapsis and to differentiate spermatocytes at various stages of meiotic prophase. Scale bar, 10 μm. Full size image Localization of the BRCA1–A complex does not rely on RNF8 Similar to RAD18, RAP80 also localizes to DNA damage sites through recognition of RNF8-dependent ubiquitin chains in somatic cells [22] , [23] , [24] . But unlike RAD18 that spreads over the sex chromosome, RAP80 is localized specifically to the unsynapsed axes in wild-type spermatocytes ( Fig. 3a ). Interestingly, the localization of RAP80 was still preserved in the Rnf8 knockout spermatocytes ( Fig. 3a ). These results suggest that the regulation of RAD18 and RAP80 is different in spermatocytes. RAP80 belongs to a big complex containing BRCA1 in somatic cells known as the BRCA1–A complex [25] , [26] , [27] , and RAP80 is required for targeting this complex to the DNA damage sites in somatic cells. To examine if RAP80 belongs to the same BRCA1–A complex in spermatocytes, we determined the localizations of other members of this complex, including BRCA1, CCDC98 and MERIT40, in spermatocytes. Consistent with our previous observation, BRCA1 localized specifically to the unsynapsed axes, and the localization was not affected by RNF8 deficiency ( Fig. 3b ). Interestingly, both CCDC98 and MERIT40 also localized to the unsynapsed axes in both wild-type and Rnf8 knockout spermatocytes ( Fig. 3c ). Although we did not check the localizations of BRCC36 and BRCC45, due to unavailability of antibodies, our observations suggest that the same BRCA1–A complex exists in spermatocytes and its members localize at the unsynapsed axes in spermatocytes. Unlike the DDR in somatic cells, the localization of BRCA1–A complex members is independent of RNF8. This suggests that the BRCA1–A complex does not recognize RNF8-dependent ubiquitin chains in spermatocytes by RAP80, as it does during DDR in somatic cells. The BRCA1–A complex is known to promote homologous recombination repair by recruiting RAD51 to DNA damage sites in somatic cells [28] . Consistent with the localization of the BRCA1–A complex, RAD51 was exclusively located at the unsynapsed axes ( Fig. 3e ). Interestingly, although RNF8 regulates the localization of RAD51 to DNA damage sites in somatic cells [29] , it had no impact on the localization of RAD51 at the unsynapsed axes in spermatocytes ( Fig. 3e ). These observations suggest that RNF8 is dispensable for homologous recombination repair of the sex chromosomes, which is likely mediated by the BRCA1–A complex and RAD51. 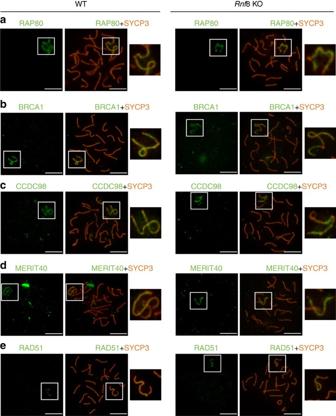Figure 3: RNF8 is dispensable for the localization of the BRCA1–A complex. Spermatocytes at pachynema from WT andRnf8knockout mice were stained using the antibodies against RAP80 (a), BRCA1 (b), CCDC98 (c), MERIT40 (d) and RAD51 (e). SYCP3 was used to visualize the chromosome synapsis and to differentiate spermatocytes at various stages of meiotic prophase. White boxes indicate the positions of the unsynapsed axes of sex chromosomes, and are magnified on the right. Scale bar, 10 μm. Figure 3: RNF8 is dispensable for the localization of the BRCA1–A complex. Spermatocytes at pachynema from WT and Rnf8 knockout mice were stained using the antibodies against RAP80 ( a ), BRCA1 ( b ), CCDC98 ( c ), MERIT40 ( d ) and RAD51 ( e ). SYCP3 was used to visualize the chromosome synapsis and to differentiate spermatocytes at various stages of meiotic prophase. White boxes indicate the positions of the unsynapsed axes of sex chromosomes, and are magnified on the right. Scale bar, 10 μm. Full size image As the BRCA1–A complex is also regulated by H2AX and MDC1, two proteins upstream of RNF8 in the DDR in somatic cells, we wondered if the BRCA1–A complex is still regulated by H2AX and MDC1 in spermatocytes. Interestingly, BRCA1 still localized at the unsynapsed axes in H2ax and Mdc1 knockout spermatocytes ( Fig. 4a ). Moreover, the localizations of RAP80, CCDC98 and MERIT40 at unsynapsed axes were also preserved in H2ax and Mdc1 knockout spermatocytes ( Fig. 4b–d ). These observations suggest that the accumulation of the BRCA1–A complex at the unsynapsed axes occurs through other mechanisms. 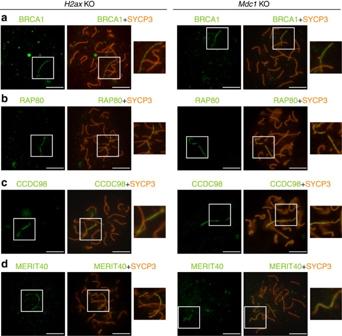Figure 4: H2AX and MDC1 are dispensable for the localization of the BRCA1–A complex. Spermatocytes at pachynema fromH2axandMdc1knockout mice were stained using the antibodies against BRCA1 (a), RAP80 (b), CCDC98 (c) and MERIT40 (d). SYCP3 was used to visualize the chromosome synapsis and to differentiate spermatocytes at various stages of meiotic prophase. White boxes indicate the positions of the unsynapsed axes of sex chromosomes, and are magnified on the right. Scale bar, 10 μm. Figure 4: H2AX and MDC1 are dispensable for the localization of the BRCA1–A complex. Spermatocytes at pachynema from H2ax and Mdc1 knockout mice were stained using the antibodies against BRCA1 ( a ), RAP80 ( b ), CCDC98 ( c ) and MERIT40 ( d ). SYCP3 was used to visualize the chromosome synapsis and to differentiate spermatocytes at various stages of meiotic prophase. White boxes indicate the positions of the unsynapsed axes of sex chromosomes, and are magnified on the right. Scale bar, 10 μm. Full size image BRCA1’s localization relies on BRCT domain To gain more insight into the mechanism by which BRCA1 localizes to the unsynapsed axes in spermatocytes, we examined if it localizes through its BRCT domains, as it does at DNA damage sites in somatic cells [30] . The BRCA1 BRCT domain is a phospho-binding module [30] . To study if the BRCA1 BRCT domain could still function as a phospho-binding module in spermatocytes, we developed a novel in vitro binding method to examine the protein localization in spermatocytes. Recombinant glutathione S- transferase (GST)-tagged BRCA1 BRCT domain was incubated with the spermatocyte spread, and the localization of the BRCA1 BRCT domain in spermatocytes was then visualized by immunostaining using an anti-GST antibody. While GST alone, a negative control, could not be observed in spermatocytes ( Fig. 5a ), the BRCA1 BRCT domain clearly localized at the unsynapsed axes ( Fig. 5b ). In addition, the localization of the recombinant BRCA1 BRCT domain at unsynapsed axes could be observed in H2ax knockout, Mdc1 knockout and Rnf8 knockout spermatocytes ( Fig. 5c ). This fully recapitulated the pattern of endogenous BRCA1 in these cells. To examine if the localization of BRCA1 requires the presence of phosphorylated proteins at the unsynapsed axes, we pretreated the spermatocyte spread with lambda phosphatase before incubating it with the recombinant BRCA1 BRCT domain. Lambda phosphatase specifically abolished the protein phosphorylation at the unsynapsed axes, including CCDC98 phosphorylation, after the pretreatment ( Fig. 5d ). Although RAP80, which localizes to the unsynapsed axes in a phosphorylation-independent manner, remained at the unsynapsed axes ( Fig. 5f ), the recombinant BRCA1 BRCT domain could no longer localize to the unsynapsed axes following phosphatase treatment ( Fig. 5g ). Consistent with this observation, mutations of the key amino acids in the phospho-binding pocket of BRCA1 BRCT domain (S1655A or K1702A) completely abolished its localization to the unsynapsed axes ( Fig. 5h ). Together, these results suggest that the recruitment of BRCA1 to the unsynapsed axes is indeed through binding of phosphorylated proteins using its BRCT domains. 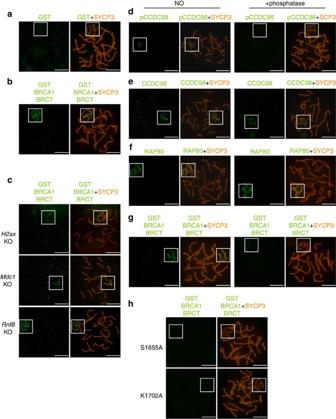Figure 5: The localization of BRCA1 relies on BRCT domain recognition. (a,b) Surface spreads of spermatocytes from WT mice were incubated with GST-tagged recombinant proteins as indicated, and stained using antibodies against GST. (c) Surface spreads of spermatocytes fromH2ax,Mdc1andRnf8knockout mice were incubated with GST-tagged BRCA1 BRCT domain proteins, and stained using antibodies against GST. (d,f) Surface spreads of spermatocytes from WT mice were treated with or without lambda protein phosphatase (phosphatase), and stained using the antibodies as indicated. (g) Surface spreads of spermatocytes from WT mice were treated with or without lambda protein phosphatase (phosphatase), incubated with GST-tagged BRCA1 BRCT domain proteins, and stained using antibodies against GST. (h) Surface spreads of spermatocytes from WT mice were incubated with GST-tagged recombinant proteins as indicated, and stained using antibodies against GST. In all panels, SYCP3 was used to visualize the chromosome synapsis and to differentiate spermatocytes at various stages of meiotic prophase. White boxes indicate the positions of the unsynapsed axes of sex chromosomes. Scale bar, 10 μm. Figure 5: The localization of BRCA1 relies on BRCT domain recognition. ( a , b ) Surface spreads of spermatocytes from WT mice were incubated with GST-tagged recombinant proteins as indicated, and stained using antibodies against GST. ( c ) Surface spreads of spermatocytes from H2ax , Mdc1 and Rnf8 knockout mice were incubated with GST-tagged BRCA1 BRCT domain proteins, and stained using antibodies against GST. ( d , f ) Surface spreads of spermatocytes from WT mice were treated with or without lambda protein phosphatase (phosphatase), and stained using the antibodies as indicated. ( g ) Surface spreads of spermatocytes from WT mice were treated with or without lambda protein phosphatase (phosphatase), incubated with GST-tagged BRCA1 BRCT domain proteins, and stained using antibodies against GST. ( h ) Surface spreads of spermatocytes from WT mice were incubated with GST-tagged recombinant proteins as indicated, and stained using antibodies against GST. In all panels, SYCP3 was used to visualize the chromosome synapsis and to differentiate spermatocytes at various stages of meiotic prophase. White boxes indicate the positions of the unsynapsed axes of sex chromosomes. Scale bar, 10 μm. Full size image It has been shown that phospho-dependent binding of CCDC 98 in the BRCA1–A complex is required for targeting BRCA1 to DNA damage sites in somatic cells [22] , [31] , [32] . We wondered if the same mechanism is used for targeting BRCA1 to the unsynapsed axes. We examined mice deficient for RAP80, which is known to be required for targeting the BRCA1–A complex to DNA damage sites through recognition of protein ubiquitination in somatic cells [33] . Rap80 knockout mice are fertile and display no defect in meiotic progression. Analysis of Rap80 knockout spermatocytes revealed that CCDC98 is absent from the unsynapsed axes of the XY body ( Fig. 6a ), but interestingly BRCA1 is still preserved ( Fig. 6b ). This suggests that the BRCA1–A complex is dispensable for targeting BRCA1 to the unsynapsed axes. It is possible that BRCA1 is targeted to the unsynapsed axes by other proteins, and that the BRCA1–A complex is tethered there through BRCA1. This is consistent with the observation that loss of ubiquitination in Rnf8 knockout spermatocytes does not affect the localization of the BRCA1–A complex ( Fig. 3a–d ). To search for other mechanisms for targeting BRCA1 to the unsynapsed axes in a phospho-dependent manner, we analysed the localizations of two other known somatic BRCA1 phospho-dependent binding partners: BACH1 from the BRCA1–B complex [30] , and CTIP from the BRCA1–C complex [34] , [35] . Interestingly, although BACH1 was not detected in the XY body ( Fig. 6c ), CTIP was specifically localized to the unsynapsed axes of the XY body ( Fig. 6d ). The localization of CTIP was not altered in H2ax , Mdc1 , Rnf8 or Rap80 knockout mice ( Fig. 6e ), which fully coincide with the localizations of BRCA1 in these mice. As direct evaluation of the impact of the loss of CTIP on the localization of BRCA1 could not be performed due to the embryonic lethality of Ctip knockout mice [36] , it is not clear if CTIP has any roles in targeting BRCA1 to the unsynapsed axes of the XY body. 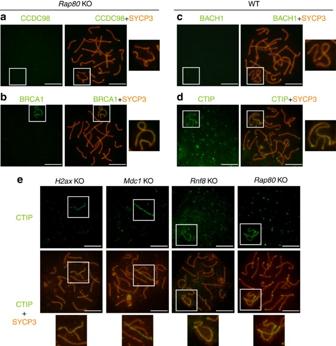Figure 6: The localization of BRCA1 does not require the BRCA1–A complex. Spermatocytes at pachynema from WT andH2ax,Mdc1,Rnf8andRap80knockout mice were stained using the antibodies against CCDC98 (a), BRCA1 (b), BACH1 (c) and CTIP (d,e). SYCP3 was used to visualize the chromosome synapsis and to differentiate spermatocytes at various stages of meiotic prophase. White boxes indicate the positions of the unsynapsed axes of sex chromosomes, and are magnified on the right. Scale bar, 10 μm. Figure 6: The localization of BRCA1 does not require the BRCA1–A complex. Spermatocytes at pachynema from WT and H2ax , Mdc1 , Rnf8 and Rap80 knockout mice were stained using the antibodies against CCDC98 ( a ), BRCA1 ( b ), BACH1 ( c ) and CTIP ( d , e ). SYCP3 was used to visualize the chromosome synapsis and to differentiate spermatocytes at various stages of meiotic prophase. White boxes indicate the positions of the unsynapsed axes of sex chromosomes, and are magnified on the right. Scale bar, 10 μm. Full size image ATM and DNAPK localize to unsynapsed axes of sex chromosomes As protein phosphorylation is important for BRCA1 localization to the unsynapsed axes independent of H2AX-MDC1-RNF8 signalling, we wondered which protein kinases are responsible for the protein phosphorylation located at the unsynapsed axes. ATR is a protein kinase that is known to localize to the unsynapsed axes [4] . Besides ATR, ATM and DNAPK are two other important protein kinases for the DDR in somatic cells and are autophosphorylated when they are activated. We examined the localizations of the active forms of these two kinases and found that both of them localized at the unsynapsed axes ( Fig. 7a ). Interestingly, the localizations of all these three protein kinases were still preserved in spermatocytes lacking H2AX, MDC1 or RNF8 ( Fig. 7a ). As the activations of ATM and DNAPK at DNA damage sites require proper H2AX-MDC1-RNF8 signalling in somatic cells [37] , [38] , this observation suggests that the regulation of these kinases at the unsynapsed axes is different from that in somatic DDR. Future studies will reveal their precise roles at the unsynapsed axes. 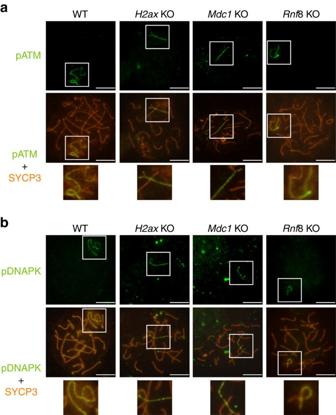Figure 7: ATM and DNAPK localize to the unsynapsed axes of sex chromosomes. Spermatocytes at pachynema from WT andH2ax,Mdc1andRnf8knockout mice were stained using the antibodies against activated phosphorylated ATM (a) and activated phosphorylated DNAPK (b). SYCP3 was used to visualize the chromosome synapsis and to differentiate spermatocytes at various stages of meiotic prophase. White boxes indicate the positions of the unsynapsed axes of sex chromosomes, and are magnified on the bottom. Scale bar, 10 μm. Figure 7: ATM and DNAPK localize to the unsynapsed axes of sex chromosomes. Spermatocytes at pachynema from WT and H2ax , Mdc1 and Rnf8 knockout mice were stained using the antibodies against activated phosphorylated ATM ( a ) and activated phosphorylated DNAPK ( b ). SYCP3 was used to visualize the chromosome synapsis and to differentiate spermatocytes at various stages of meiotic prophase. White boxes indicate the positions of the unsynapsed axes of sex chromosomes, and are magnified on the bottom. Scale bar, 10 μm. Full size image Many proteins in the DDR pathways accumulate in the XY body of spermatocytes at pachynema. This suggests that the DNA breaks are not yet repaired on the sex chromosomes. The delay of the repair might be caused by the fact that the sex chromosomes do not have homologous chromosomes, which are favourable templates for homologous recombination repair during meiotic prophase. The DNA breaks on the sex chromosomes are likely to be repaired by homologous recombination using their sister chromatids instead, which is not preferred and used as a back-up at the later stage of meiotic prophase. During this inefficient repair process in the XY body, transcription on the sex chromosomes is silenced, which is known as MSCI (ref. 2 ). Although the mechanism is not clear, it is likely that MSCI is similar to DNA damage-induced transcriptional silencing in somatic cells [39] , which is a protective measure downstream of the DDR to prevent the generation of truncated RNA. Although many DDR proteins accumulate in the XY body, it is puzzling why some proteins are restricted to the unsynapsed axes while others spread over the sex chromosomes. This unique feature might be a result of the prolonged presence of DNA damage in the XY body. It has been shown that the localization of proteins to the unsynapsed axes is independent of canonical H2AX-MDC1 signalling [3] , [4] . In this study, we have identified several new proteins that are restricted to the unsynapsed axes, and their localization is not regulated by H2AX-MDC1-RNF8 pathways either. This is reminiscent of the observations in somatic cells that the localization of some proteins to the DNA damage sites at early time points is independent of H2AX, MDC1 or RNF8 (refs 40 , 41 ). It is, therefore, possible that similar mechanisms for protein recruitment are shared between these two events. Previous studies have shown that ATR is localized at the unsynapsed axes. Interestingly, we observed the localization of two other DDR-related protein kinases (ATM and DNAPK) at the unsynapsed axes. This suggests that protein phosphorylation is indeed important for the DDR signalling at unsynapsed axes. Recent studies suggest that these protein kinases at the unsynapsed axes are also regulated by proteins containing the HORMA domain, which preferentially associate with unsynapsed chromosomes and are likely to contribute to the initiation of the DDR on the unsynapsed axes of the XY body [42] , [43] , [44] , [45] , [46] . In agreement with this, BRCA1 is likely to be recruited through binding to phosphorylated proteins. As BRCA1 is upstream of the localization of ATR to unsynapsed axes [47] , [48] , it is likely that ATM and/or DNAPK-dependent protein phosphorylation recruits BRCA1 to the unsynapsed axes. The identity of the phosphorylated protein remains to be found. Besides the proteins enriched at the unsynapsed axes, other DDR proteins spread over the sex chromosomes. This is similar to the observation in somatic cells that DDR proteins spread megabases away from the actual DNA breaks [49] . The spread of DDR proteins over the sex chromosomes explains why the whole sex chromosomes, but not only the regions at the unsynapsed axes, are transcriptionally silenced. Based on the observation that DDR proteins no longer spread over the sex chromosomes in Mdc1 knockout spermatocytes, it was suggested that H2AX and MDC1 control the spread of DDR proteins over the whole sex chromosomes despite the fact that they are dispensable for the signalling on the unsynapsed axes [4] . However, as Mdc1 knockout spermatocytes arrest at mid-pachynema without proper formation of the XY body, it is difficult to distinguish if the defective spreading of DDR proteins to the sex chromosomes is due to the absence of MDC1’s function in the DDR signalling or the absence of XY body where the spreading takes place. In this respect, Rnf8 knockout spermatocytes are more suitable for studying the DDR signalling over the sex chromosomes, as there is no defect in meiotic progression and the XY body readily forms at pachynema in Rnf8 knockout spermatocytes. Using Rnf8 knockout spermatocytes, we found that the DDR signalling of the sex chromosome is largely similar to the DDR signalling in somatic cells. The proteins upstream of RNF8 (H2AX and MDC1) are retained and those downstream of RNF8 (K63-Ub, K48-Ub, 53BP1 and RAD18) are absent in Rnf8 knockout spermatocytes. Differences were also noticed between the signalling pathways in spermatocytes and somatic cells. For example, protein sumoylation is not dependent on RNF8 in spermatocytes, which is consistent with the observation that sumoylation precedes H2AX phosphorylation in the XY body [50] . It has been shown that the modifications by SUMO1 and SUMO2/3 mainly occur on BRCA1 and 53BP1, respectively, during the DDR in somatic cells [12] , [13] . As BRCA1 does not localize over the whole sex chromosomes and the spread of 53BP1 over sex chromosomes is absent in Rnf8 knockout spermatocytes, it is likely that the modifications by SUMO1 and SUMO2/3 on sex chromosomes predominantly occur on other proteins, which remain to be identified in spermatocytes. In summary, we have studied the regulation of DDR signalling in the XY body of spermatocytes at pachynema. In our model, some proteins are recruited to the unsynapsed axes independent of canonical DDR pathways. The DDR then spreads over the whole sex chromosomes by amplification of γH2AX-MDC1-RNF8 signalling, which recruits another set of proteins ( Fig. 8 ). We have also found that Rnf8 knockout mice are invaluable tools for studying meiotic DDR. In addition, we have generated a novel in vitro binding method for analysing DDR proteins, which allows easy visualization of DDR proteins at the XY body while circumventing the need for antibodies against these proteins. 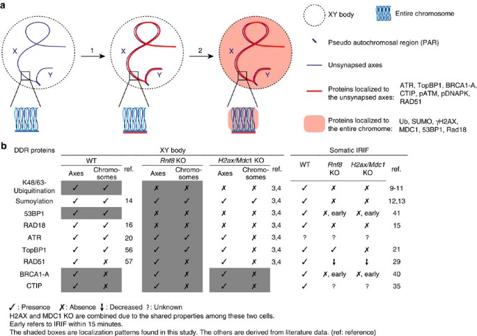Figure 8: DDR at the XY body and at somatic DNA damage sites are different. (a) Model of the DDR in the XY body. Some proteins are directly recruited to the unsynapsed axes independent of canonical DDR pathways. The DDR then spreads over the sex chromosomes by amplification of γH2AX-MDC1-RNF8 signalling, which recruits another set of proteins. (b) Summary of the localizations of DDR proteins in XY body at meiotic prophase and their formations of ionizing radiation-induced foci (IRIF) in somatic cells. Figure 8: DDR at the XY body and at somatic DNA damage sites are different. ( a ) Model of the DDR in the XY body. Some proteins are directly recruited to the unsynapsed axes independent of canonical DDR pathways. The DDR then spreads over the sex chromosomes by amplification of γH2AX-MDC1-RNF8 signalling, which recruits another set of proteins. ( b ) Summary of the localizations of DDR proteins in XY body at meiotic prophase and their formations of ionizing radiation-induced foci (IRIF) in somatic cells. Full size image Mice Animal studies were ethically approved by the University Committee on Use and Care of Animals of the University of Michigan. Rnf8 and Rap80 knockout mice were reported previously [7] , [33] . H2ax and Mdc1 knockout mice are from Andre Nussenzweig and Zhenkun Lou, respectively. All of the mice were housed in an AAALAC accredited facility in accordance with the National Research Council’s guide for the care and use of laboratory animals. Immunofluorescence staining Immunofluorescence staining (IF) was performed at room temperature. The slides were first blocked with IF buffer (5% goat serum in PBS) for 0.5 h before incubating with primary antibodies diluted in IF buffer for 1 h. The slides were then washed three times with PBS and incubated with secondary antibodies (1:1,000) diluted in IF buffer for 0.5 h. The slides were subsequently washed three times with PBS and mounted with coverslips. All images were taken using Olympus IX71 microscope. All secondary antibodies (FITC (fluorescein isothiocyanate) or TRITC (tetramethyl rhodamine isothiocyanate)-labelled goat-anti-mouse/rabbit IgG) were from Jackson ImmunoResearch. Primary antibodies were used at 1:1,000 dilutions unless otherwise indicated. The following antibodies were previously described: ATR [51] , TopBP1 (ref. 52 ), RAP80, BRCA1 (ref. 33 ), CCDC98 (1:100) (ref. 32 ), pCCDC98 (1:100) (ref. 32 ), MERIT40 (1:100) (ref. 53 ), 53BP1 (ref. 18 ), RAD51 (ref. 54 ), and BACH1 (1:100) (ref. 30 ). The following antibodies were purchased: ubiquitin (FK2) (Millipore, 04-263), SUMO1 (1:200, Invitrogen, 33-2400), γH2AX (Millipore, 05-636), RAD18 (1:500, Proteintech, 18333-1-AP), pATM (1:200, Cell Signaling, 4526), rabbit against SYCP3 (Novus, NB300-232), and mouse against SYCP3 (Abcam, ab97672). The following antibodies were kind gifts from others: K48-Ub (Genentech), K63-Ub (Genentech), SUMO2/3 (1:200, Michael Matunis), MDC1 (1:100, Zhenkun Lou), CTIP (1:50, Richard Baer), and pDNAPK (1:50, David Chen). Antibodies against GST (1:1,000) were generated using the full length GST protein. The specificities of the following antibodies were well established: anti-ubiquitin (FK2) (ref. 55 ), K48-Ub (ref. 8 ) and K63-Ub (ref. 8 ). The specificities of the following antibodies were confirmed as they have the same staining patterns as shown in the literature using other antibodies that recognize the same proteins: anti-SYCP3 (ref. 47 ), SUMO1 (ref. 50 ), SUMO2/3 (ref. 50 ), γH2AX (ref. 3 ), MDC1 (ref. 4 ), RAD18 (ref. 16 ), ATR (ref. 47 ), TopBP1 (ref. 56 ), BRCA1 (ref. 47 ) and RAD51 (ref. 57 ). The specificities of the following antibodies were confirmed by loss of signals in the knockouts: anti-53BP1 (ref. 18 ), RAP80 (ref. 33 ), pATM (ref. 58 ) and pDNAPK (ref. 59 ). The specificity of anti-CTIP antibody was confirmed previously by short hairpin RNA-mediated knockdown in mouse cells [60] . The specificities of the following antibodies in detecting mouse proteins in the XY body were also confirmed by using additional antibodies that recognize the same proteins: anti-pATM (Cell Signaling, 5883), pDNAPK (Abcam, ab18356) and CTIP [34] . The specificities of anti-CCDC98 and pCCDC98 antibodies were confirmed as they recognize the same protein and have the same staining patterns in the XY body. The specificity of anti-CCDC98 antibody was further confirmed by loss of signals in the Rap80 knockout spermatocytes. The specificities of anti-MERIT40 was confirmed by the observation that recombinant MERIT40 localized to the unsynapsed axes using the in vitro binding method developed in this study. The absence of BACH1 in the XY body was also confirmed by another antibody that recognizes a different region of mouse BACH1 (Santa Cruz, sc-365708). Surface spread of spermatocytes Spermatocytes were dissociated from seminiferous tubules by collagenase treatment (1 mg ml −1 ) at 37 °C. Isolated cells were collected and incubated for 10 min in buffer containing 30 mM Tris-HCl pH 8.2, 50 mM sucrose, and 17 mM sodium citrate. The cells were then pelleted and resuspended in 100 mM sucrose before being spread onto slides pre-coated with PFA solution (1% PFA, 0.15% Triton-X-100, 10 mM sodium borate, pH 9.2). The slides were kept in a humidified chamber for 4 h, washed with 0.4% Photoflo (Kodak), and dried. In vitro binding of recombinant proteins to spermatocytes GST-tagged proteins were expressed in BL21 bacteria, purified using glutathione sepharose, and dialyzed with 1 × PBS. Ten nanomolar of recombinant protein was added to the slides with surface spread of spermatocytes, and incubated for 1 h in room temperature. The excess protein was then removed and the slides were washed three times with 1 × PBS before subjected to immunofluoresence staining using antibodies against GST. To remove phosphate groups from proteins in the surface spread of spermatocytes, each slide was treated with 1,000 units of lambda protein phosphatase (NEB) for 1 h at room temperature in the buffer provided by the supplier. How to cite this article: Lu, L. -Y et al . Regulation of the DNA damage response on male meiotic sex chromosomes. Nat. Commun. 4:2105 doi: 10.1038/ncomms3105 (2013).